p53 and p16INK4Aindependent induction of senescence by chromatin-dependent alteration of S-phase progression Senescence is triggered by various cellular stresses that result in genomic lesions and DNA damage response activation. However, the role of chromatin and DNA replication in senescence induction remains elusive. Here we show that downregulation of p300 histone acetyltransferase activity induces senescence by a mechanism that is independent of the activation of p53, p21 CIP1 and p16 INK4A . This inhibition leads to a global H3, H4 hypoacetylation, initiating senescence-associated heterochromatic foci formation during S phase, together with a global decrease in replication fork velocity, and alteration of DNA replication timing. This replicative stress occurs without DNA damage and checkpoint activation, but results in a robust G2/M cell cycle arrest, within only one cell cycle. These results provide new insights into the control of S-phase progression by p300, and identify an unexpected chromatin-dependent alternative mechanism for senescence induction, which could possibly be exploited to treat cancer by senescence induction without generating further DNA damage. Cellular senescence is characterized by a stable cell cycle arrest that is triggered by various forms of stress stimuli including oncogene activation (oncogene-induced senescence, OIS) or telomere shortening (replicative senescence), and is considered as a barrier to tumourigenesis [1] . This arrest depends on the activation of the cyclin-dependent kinase (CDK) inhibitors (p21 CIP1 and p16 INK4A ), components of the tumour-suppressor pathways that are governed by the p53 and retinoblastoma (pRB) proteins, respectively [2] . Activation of the DNA damage response (DDR), triggered by DNA single-strand and/or double-strand breaks, has been described as a common feature of telomere-initiated or OIS [3] , [4] . Moreover, dramatic changes in chromatin structure seem to contribute to the irreversible nature of the senescent state, especially through the formation of senescence-associated heterochromatic foci (SAHF), which are characterized by hypoacetylation of histones, tri-methylation of histone H3 on lysine 9 (H3K9me3) and the presence of facultative heterochromatin proteins [5] , [6] , [7] . Chromatin organization is partly regulated by the balance of activity between histone acetyltransferases (HATs) and histone deacetylases. The HAT p300, which is involved in the regulation of cellular growth, differentiation and survival, can directly modify the chromatin state and interact with complexes that mediate chromatin metabolism [8] , [9] . We therefore decided to study the role of p300 in senescence induction. Here demonstrate that repression of p300 HAT activity, which induces global histone H3 and H4 hypoacetylation, initiates SAHF formation during S phase. This inhibition leads to a senescence-like growth arrest in G2/M, within only one cell cycle. Interestingly, we observed an alteration in the replication activity characterized by a global decrease in replication fork velocity, and a change in DNA replication timing, occurring in the absence of DNA damage and checkpoint activation. Finally, we show that the downregulation of p300 HAT activity leads to p53, p21 CIP1 and p16 INK4A -independent senescence. These results reveal an unexpected and new mechanism for senescence induction involving inhibition of p300 activity. Our findings suggest that chromatin-dependent alteration can robustly induce senescence without activation of the commonly associated senescence pathways. Inhibition of p300 HAT activity induces senescence We used two short hairpin RNAs (shp300-1 and shp300-2) to stably inhibit p300 expression in the hTERT-immortalized human diploid fibroblast (HDF) cell line TIG3(et). In response to reduced p300 expression, we observed the upregulation of the CDK inhibitors p16 INK4A and p21 CIP1 , an increase in senescence-associated β-galactosidase (SA-β-Gal) activity and SAHF formation ( Fig. 1a–c ). These changes are hallmarks of cellular senescence [2] . Assuming that cellular senescence can be triggered by different stresses, including oncogene activation or telomere shortening [2] , we wondered whether inactivation of p300 activity also occurs in these types of cellular senescence and may participate in cell cycle arrest. Interestingly, we observed a dramatic decrease in p300 expression levels in HDF cells in which premature senescence was induced by overexpressing the oncogene Ras V12 ( Supplementary Fig. S1a,b ). Similarly, induction of replicative senescence on serial passaging in non-immortalized fibroblasts also lead to a strong decrease in p300 expression ( Supplementary Fig. S1c,d ). Finally, we did not observe downregulation of p300 expression in quiescent cells ( Fig. 1a ), suggesting that downregulation of p300 might be a common event specifically associated with the senescence induction process. 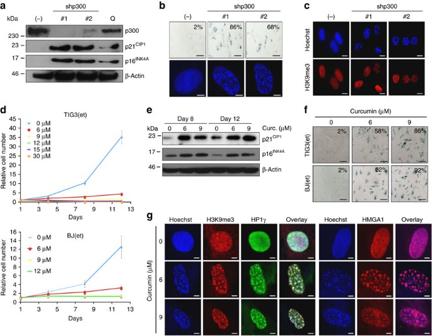Figure 1: Inhibition of p300 HAT activity induces senescence. (a–c) Stable downregulation of p300 by expression of two distinct shRNAs #1, #2 in TIG3(et) cells. Cells were collected and stained 12 days after selection. (a) Immunoblot analysis with β-actin as a loading control and Q for quiescent cells. (b) Images of SA-β-gal-stained (upper panel) and Hoechst-stained (lower panel) cells to detect SAHF. Scale bars are equal to 5 μm. (c) Images of a large field with H3K9me3 and Hoechst staining to detect SAHF. Scale bars are equal to 10 μm. (d–g) TIG3(et) and BJ(et) cells treated with different doses of curcumin or vehicle (0) as control. (d) Analysis by proliferation curve. Means of three experiments with standard deviation. (e) Immunoblot analysis with β-actin as a loading control for TIG3(et) cells. (f–g) Cells were collected and stained 12 days after selection. (f) SA-β-gal activity. Scale bars are equal to 40 μm. (g) Immunofluorescence analysis with specific antibodies for co-localization with SAHF for TIG3(et) cells. Scale bars are equal to 5 μm. (b,f) Percentage of SA-β-gal-positive cells is indicated in insert. Figure 1: Inhibition of p300 HAT activity induces senescence. ( a – c ) Stable downregulation of p300 by expression of two distinct shRNAs #1, #2 in TIG3(et) cells. Cells were collected and stained 12 days after selection. ( a ) Immunoblot analysis with β-actin as a loading control and Q for quiescent cells. ( b ) Images of SA-β-gal-stained (upper panel) and Hoechst-stained (lower panel) cells to detect SAHF. Scale bars are equal to 5 μm. ( c ) Images of a large field with H3K9me3 and Hoechst staining to detect SAHF. Scale bars are equal to 10 μm. ( d–g ) TIG3(et) and BJ(et) cells treated with different doses of curcumin or vehicle (0) as control. ( d ) Analysis by proliferation curve. Means of three experiments with standard deviation. ( e ) Immunoblot analysis with β-actin as a loading control for TIG3(et) cells. ( f–g ) Cells were collected and stained 12 days after selection. ( f ) SA-β-gal activity. Scale bars are equal to 40 μm. ( g ) Immunofluorescence analysis with specific antibodies for co-localization with SAHF for TIG3(et) cells. Scale bars are equal to 5 μm. ( b,f ) Percentage of SA-β-gal-positive cells is indicated in insert. Full size image To obtain further insight into the mechanisms involved, we specifically inhibited the HAT activity of p300, which is the major activity of this protein responsible for acetylation of histone H3 and H4. We treated the HDF TIG3(et) cells for 12 days with increasing doses of curcumin, a potent inhibitor of p300 HAT activity [10] . We observed a proliferation arrest even at low doses (<12 μM) ( Fig. 1d ). This cell cycle arrest was associated with the upregulation of CDK inhibitors, p16 INK4A , and p21 CIP1 , an increase in SA-β-Gal activity and formation of SAHF, which co-localized with HP1γ, H3K9me3 and HMGA1, as previously described [6] ( Fig. 1e,f,g ). We confirmed these results in another hTERT-immortalized HDF cell line, BJ(et) ( Fig. 1d and f ), demonstrating that inhibition of p300 HAT activity by curcumin induces premature senescence in HDF, thus recapitulating the effects of p300 downregulation. To further confirm that inhibition of p300 HAT activity is involved in senescence induction, we used CTPB, a specific activator of p300 activity [10] . CTPB treatment prevented curcumin-induced senescence in HDF cells, as observed by the rescue of their proliferation rate and the decrease in SAHF formation ( Supplementary Fig. S2 ), confirming that inhibition of p300 HAT activity is required for senescence induction. Moreover, the use of C646, another specific inhibitor of p300 HAT activity [11] , confirmed that inhibition of p300 HAT activity induces SAHF formation and senescence-like growth arrest, when compared with the inactive form C37 ( Supplementary Fig. S3 ). Together these results demonstrate that the specific loss of p300 HAT activity can induce cellular senescence. SAHF-dependent G2/M arrest within one cell cycle To further elucidate the mechanism of this senescence-associated growth inhibition, we analysed the cell cycle profile of HDF cells in the presence of curcumin by FACS. Surprisingly, a 72-h curcumin treatment gave rise to an accumulation of cells in G2/M phase, when comapared with mock-treated cells (6.5% versus 26.6%, respectively) whereas no change in G1 phase proportion was observed (63.4% versus 65.4%, respectively) ( Fig. 2a ). This contrasts with the common cell cycle arrest of senescent fibroblasts that is usually observed in G1 phase [2] . Assuming that the senescence phenotype generally accumulates progressively over multiple cell cycles [4] , we tested the effect of p300 HAT inhibition on the cell cycle over time. We synchronized cells in G0/G1 by serum starvation and released them in the presence of shp300-1 (hereafter TIG3(et)/p300kd HDF cells). Interestingly, 72 h after the release, we also observed an accumulation of cells in G2/M phase, demonstrating that the inhibition of p300 triggers this cell cycle arrest ( Fig. 2b ). Similarly, synchronized cells, released in the presence of curcumin, accumulate at the G2/M transition in a dose-dependent manner ( Fig. 2c ). Finally, to formally show that the cells enter senescence in one cell cycle, we pulse-labelled HDF cells with a nucleotide analogue EdU at the beginning of S phase (16 h after the serum release). Remarkably, two weeks after the EdU pulse labelling, curcumin-treated cells retained a staining pattern identical to that observed in the 1 h post-labelling control, whereas control-treated cells were no longer labelled. This indicates that the treated cells were stably arrested in their first cell cycle ( Fig. 2d ). Together, these results show that p300 HAT inhibition induces a G2/M block in HDF cells that leads to a senescence-like growth arrest within one cell cycle. 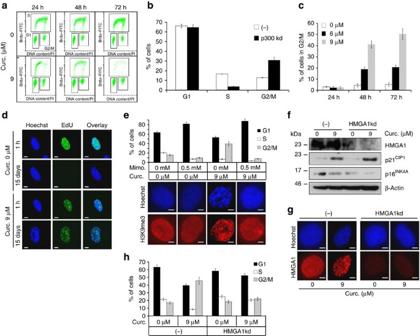Figure 2: Inhibition of p300 HAT induces a SAHF-dependent senescence G2/M cell cycle arrest within one cell cycle. (a) Cell cycle distribution of curcumin-treated or vehicle (0) as control non-synchronized TIG3(et) cell population analysed by FACS at different time points of treatment. (b) Synchronized TIG3(et) cells in G0 by serum starvation during 5 days with medium containing 0.5% FBS, then released in 10% FBS medium in presence of shp300-1 or empty vector (−) as control and analysed by FACS 72 h after serum release for cell cycle distribution. (c) Synchronized TIG3(et) cells in G0 by serum starvation, released in presence of 6 and 9 μM curcumin (Curc.) or vehicle (0) as control, and analysed by FACS at different time points after release, for cell cycle distribution. (d) Immunofluorescence of EdU pulse-labelled TIG3(et) cells for 1 hour, 16 hours after serum release in presence of curcumin or vehicle (0) as control and analysed at the indicated times. (e) TIG3(et) cells were synchronized by serum starvation, released in serum in presence or absence of 9 μM curcumin (Curc.) and in presence or absence of 0.5 mM mimosine (Mimo.). Cells were collected 72 h after release and analysed by FACS (upper panel) for cell cycle distribution and by immunofluorescence (lower panel) to detect SAHF. (f–h) Synchronized TIG3(et)/HMGA1kd and TIG3(et)/(−) (for empty vector) cells in G0 by serum starvation, then released in 10% FBS medium in presence of 9 μM curcumin for 72 h. (f) Immunoblot analysis with β-actin as a loading control. (g) Immunofluorescence analysis with specific antibodies for co-localization with SAHF. (h) FACS analysis for cell cycle distribution. (b,c,e,h) Shown are the results of two independent experiments performed in duplicate. Error bars show the range. (d,e,g) Scale bars are equal to 5 μm. Figure 2: Inhibition of p300 HAT induces a SAHF-dependent senescence G2/M cell cycle arrest within one cell cycle. ( a ) Cell cycle distribution of curcumin-treated or vehicle (0) as control non-synchronized TIG3(et) cell population analysed by FACS at different time points of treatment. ( b ) Synchronized TIG3(et) cells in G0 by serum starvation during 5 days with medium containing 0.5% FBS, then released in 10% FBS medium in presence of shp300-1 or empty vector (−) as control and analysed by FACS 72 h after serum release for cell cycle distribution. ( c ) Synchronized TIG3(et) cells in G0 by serum starvation, released in presence of 6 and 9 μM curcumin (Curc.) or vehicle (0) as control, and analysed by FACS at different time points after release, for cell cycle distribution. ( d ) Immunofluorescence of EdU pulse-labelled TIG3(et) cells for 1 hour, 16 hours after serum release in presence of curcumin or vehicle (0) as control and analysed at the indicated times. ( e ) TIG3(et) cells were synchronized by serum starvation, released in serum in presence or absence of 9 μM curcumin (Curc.) and in presence or absence of 0.5 mM mimosine (Mimo.). Cells were collected 72 h after release and analysed by FACS (upper panel) for cell cycle distribution and by immunofluorescence (lower panel) to detect SAHF. ( f–h ) Synchronized TIG3(et)/HMGA1kd and TIG3(et)/(−) (for empty vector) cells in G0 by serum starvation, then released in 10% FBS medium in presence of 9 μM curcumin for 72 h. ( f ) Immunoblot analysis with β-actin as a loading control. ( g ) Immunofluorescence analysis with specific antibodies for co-localization with SAHF. ( h ) FACS analysis for cell cycle distribution. ( b,c,e,h ) Shown are the results of two independent experiments performed in duplicate. Error bars show the range. ( d,e,g ) Scale bars are equal to 5 μm. Full size image Because the G2/M senescence-like growth arrest occurs within one cell cycle, we also hypothesized that S-phase progression might also be required for senescence induction by p300 HAT inhibition. To test this possibility, we co-treated curcumin-treated cells with mimosine, an inhibitor of the G1/S transition, and found that ongoing replication was necessary for SAHF formation in this context ( Fig. 2e ). Finally, we wondered whether p300 inhibition could promote a SAHF-dependent induction of senescence. We inhibited the expression of HMGA1, which is known to block SAHF formation and senescence induction [6] , with a specific shRNA. We observed that SAHF formation was required for the G2/M senescence-like growth arrest induced by inhibition of p300 HAT activity ( Fig. 2f-h ), establishing a direct link between SAHF formation and cell cycle arrest. Alteration of S-phase progression by p300 HAT inhibition Because SAHF formation is described as a multistep process involving acetylation changes of chromatin [7] , we investigated the effect of p300 inhibition on histone acetylation. Interestingly, we observed an immediate and global hypoacetylation of histones H3 and H4 in curcumin-treated and p300kd HDF cells ( Fig. 3a ), which was also prevented by CTPB, the specific activator of p300 HAT activity ( Fig. 3b ). Moreover, the chromatin loading of the minichromosome maintenance protein 7 (MCM7), a member of the pre-replicative complex, and the sliding clamp protein PCNA, were impaired, revealing that histone hypoacetylation might interfere with the DNA replication process ( Fig. 3a ). This hypoacetylation was followed by a rapid accumulation of SAHF after release in the presence of curcumin in more than 50% of cells 48 h after treatment. This indicates that SAHF initiate during the S phase preceding the G2/M block, as confirmed by the presence of SAHF during ongoing DNA synthesis ( Fig. 3c ). 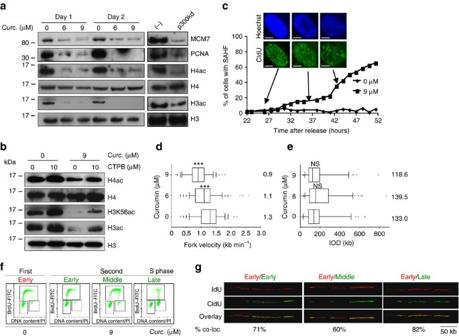Figure 3: Alteration of S-phase progression by inhibition of p300 HAT activity. (a–g) Synchronized TIG3(et) cells in G0 by serum starvation during 5 days with medium containing 0.5% FBS, then released in 10% FBS medium and treated as follows. (a) Cells treated with curcumin (Curc.) (left panel) or infected with shp300-1 (right panel). Vehicle (0) or empty vector (−) as control. Immunoblot of chromatin extracts at the indicated time points with histone H3 as a loading control. (b) Immunoblot of chromatin extracts from cells co-treated with curcumin and CTPB or vehicle as control for 24 h. (c) Time course experiment of SAHF formation in curcumin-tretated cells or vehicle (0). In insert, representative immunofluorescence of CldU and Hoechst staining to detect SAHF during S-phase progression in curcumin-treated cells. Scale bars are equal to 5 μm. (d-e) Curcumin-treated cells or vehicle (0) as control were successively pulse-labelled with IdU (15 min) and CldU (30 min) and analysed by DNA combing 24 h after treatment for measurement of (d) replication fork velocity (n=200) and (e) inter-origin distance (IOD), (n=100). Boxes correspond to 25–75 percentile, whiskers to 5–95 percentile and the line near within the box marks the median (50th percentile). Median values are indicated on the right. Statistical analysis was performed using unpairedttest (***P<0.0001; NS, not significant). (f,g) For replication timing studies, cells were released in 10% FBS medium and pulse labelled for 3 h with 25 μM IdU followed by a 3 h thymidine chase to label DNA at the early S phase. Cells were resynchronized by serum starvation for 5 days and released in 10% FBS medium in presence of curcumin and pulse labelled for 3 h with CldU in early, middle or late S phase. (f) Cell cycle distribution of cells during the first cell cycle (left panel) and curcumin-treated cells during the second cycle (right panel). (g) Molecular DNA combing analysis and quantification of CldU DNA regions overlapping with IdU. At least 4 Mb of fibres presenting both IdU and CldU tracks were analysed for the quantification, and percentages represent the fraction of CldU regions co-localizing with IdU. Figure 3: Alteration of S-phase progression by inhibition of p300 HAT activity. ( a–g ) Synchronized TIG3(et) cells in G0 by serum starvation during 5 days with medium containing 0.5% FBS, then released in 10% FBS medium and treated as follows. ( a ) Cells treated with curcumin (Curc.) (left panel) or infected with shp300-1 (right panel). Vehicle (0) or empty vector (−) as control. Immunoblot of chromatin extracts at the indicated time points with histone H3 as a loading control. ( b ) Immunoblot of chromatin extracts from cells co-treated with curcumin and CTPB or vehicle as control for 24 h. ( c ) Time course experiment of SAHF formation in curcumin-tretated cells or vehicle (0). In insert, representative immunofluorescence of CldU and Hoechst staining to detect SAHF during S-phase progression in curcumin-treated cells. Scale bars are equal to 5 μm. ( d - e ) Curcumin-treated cells or vehicle (0) as control were successively pulse-labelled with IdU (15 min) and CldU (30 min) and analysed by DNA combing 24 h after treatment for measurement of ( d ) replication fork velocity ( n =200) and ( e ) inter-origin distance (IOD), ( n =100). Boxes correspond to 25–75 percentile, whiskers to 5–95 percentile and the line near within the box marks the median (50th percentile). Median values are indicated on the right. Statistical analysis was performed using unpaired t test (*** P <0.0001; NS, not significant). ( f,g ) For replication timing studies, cells were released in 10% FBS medium and pulse labelled for 3 h with 25 μM IdU followed by a 3 h thymidine chase to label DNA at the early S phase. Cells were resynchronized by serum starvation for 5 days and released in 10% FBS medium in presence of curcumin and pulse labelled for 3 h with CldU in early, middle or late S phase. ( f ) Cell cycle distribution of cells during the first cell cycle (left panel) and curcumin-treated cells during the second cycle (right panel). ( g ) Molecular DNA combing analysis and quantification of CldU DNA regions overlapping with IdU. At least 4 Mb of fibres presenting both IdU and CldU tracks were analysed for the quantification, and percentages represent the fraction of CldU regions co-localizing with IdU. Full size image As S phase is tightly regulated to ensure total genome duplication and stability, we hypothesized that p300 HAT inhibition could trigger an alteration of S-phase progression by modifying chromatin status during ongoing S phase, leading to SAHF formation and G2/M arrest. To address this question, we first estimated the length of S phase in synchronized cells released in the presence of curcumin, and found a twofold increase in S-phase length when compared with untreated cells (24 h versus 12 h, respectively) ( Supplementary Fig. S4 ), suggesting a possible alteration of replication fork progression. To gain further insight into the alteration of the replication process in p300 inhibited cells, we performed in vivo DNA labelling and molecular DNA combing analysis. Interestingly, we observed a marked slowdown of the median replication fork velocity in curcumin-treated synchronized cells ( Fig. 3d ), and we obtained the same results when we analysed the replication fork velocity in non-synchronized cells, showing that p300 HAT inhibition interferes with the progression of DNA replication forks. Whereas modifications of fork progression are generally associated with activation of dormant origins [12] , we did not detect significant changes in the median inter-origin distances ( Fig. 3e ). Furthermore, we did not observe modifications in the distribution of the classified replication figures [13] in curcumin-treated cells ( Supplementary Fig. S5 ), suggesting that the increased S-phase length might not be due to replicative stress, even though we measured a doubling of S-phase length. However, we calculated that this increase in S-phase length could not be explained only by the 30% decrease in replication fork velocity (1.3 kb min −1 versus 0.9 kb min −1 , for untreated and 9 μM curcumin-treated cells, respectively), and might be partly because of an extended period of the time for replication origin cluster activation. The entire genome is replicated in a programmed manner, with specific regions undergoing DNA synthesis at different times during S phase. The histone acetylation level is one of the marks that distinguish early- and late-replicating regions. For instance, in early S phase, histones H3 and H4 embedded in chromatin are generally hyperacetylated, whereas in late S phase they are hypoacetylated [14] , [15] , regulating the time of replication origin firing [15] . We thus examined whether the observed hypoacetylation of histones induced by the curcumin-mediated inhibition of the p300 HAT activity, might be responsible for an alteration of the replication timing. To answer this question, we used our synchronized cell system and pulse-labelled the early S phase replicating DNA in the absence of curcumin and then, the early, middle or late S phase replicating DNA of the following cell cycle, in the presence of curcumin. We first confirmed the timing specificity of each S-phase population by FACS analysis ( Fig. 3f ). Then, we analysed whether the early S-phase-labelled DNA from the first cell cycle might be replicated in early, middle or late S phase in the second cell cycle after inhibition of p300 HAT by curcumin, using molecular DNA combing. Interestingly, we observed an important and similar overlap between the early-replicating DNA regions of the first S phase and each of the early-, middle- or late-replicating DNA of the second S phase ( Fig. 3g ). This indicates that regions usually defined as early replicating in normal conditions have an altered replication time following p300 inhibition. This result demonstrates that downregulation of p300 HAT activity leads to a global desynchronization of origin activation timing in S phase, as previously suggested by the progressive increase of SAHF formation preceding the G2/M block ( Fig. 3c ). Altogether, these results indicate that hypoacetylation of chromatin triggered by p300 inhibition initiates both SAHF formation and a desynchronization of the replication timing, leading to a doubling of S-phase length. p300 HAT inhibition induces senescence without DNA damage DNA damage, the primary inducer of replication fork stalling, activates the intra-S-phase checkpoint [16] . Activation of the DDR, that is triggered by DNA single-strand and/or double-strand breaks, is a common feature associated with senescence [3] , [4] . Key DDR-signalling components are the protein kinases Ataxia-telangiectasia-mutated (ATM) and Ataxia-telangiectasia and Rad3-related (ATR), which activate the downstream kinases CHK2 and CHK1, respectively, leading to a cell cycle arrest [17] . Furthermore, acetylation of histone H3 on lysine 56 (H3K56) has recently been shown to be mediated by p300 HAT activity and to have a critical role in packaging DNA into chromatin for DNA replication and repair [18] , [19] , [20] , [21] , [22] . We therefore investigated whether senescence induced by p300 HAT inhibition was also dependent on the activation of DDR. We used aphidicolin, a DNA polymerase inhibitor, as a positive control. Surprisingly, we did not detect DNA damage foci in curcumin-treated and p300kd cells at any time of the treatment, as revealed by the absence of histone variant H2AX phosphorylation (γH2AX) ( Fig. 4a ). Moreover, we did not observe the presence of DNA breaks in curcumin-treated and p300kd cells, whereas aphidicolin-treated cells harboured many DNA breaks as detected by comet assay ( Fig. 4b ). Further DDR-signalling analysis in curcumin-treated and p300kd cells revealed that protein kinases CHK1 and CHK2 were not activated, as showed by the lack of phosphorylation of serine 345 and threonine 68, respectively ( Fig. 4c ). In addition, inhibition of p300 HAT by curcumin did not lead to phosphorylation of p53 on serine 15, which is commonly associated with the DDR response. Furthermore, we observed a specific decrease in the H3K56 acetylation chromatin mark, as expected for a mechanism unrelated to DNA damage induction and DDR activation ( Fig. 4d ). Moreover, the inhibition of checkpoint activation with caffeine (1 mM) did not prevent the accumulation of curcumin-treated cells in G2/M phase ( Fig. 4e ), confirming that curcumin-induced senescence is independent of ATM and ATR activation. Interestingly, it was recently described that the Cdc25B dual specificity phosphatase, which controls the G2/M phase checkpoint by activating CDK1-Cyclin B activity, was specifically degraded in cells treated with drugs causing non-genotoxic stress, in the absence of DDR activation, leading to a G2/M cell cycle arrest [23] . 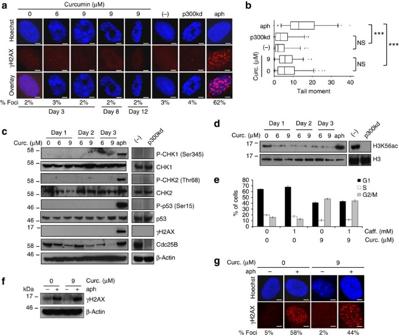Figure 4: Inhibition of p300 HAT induces senescence in absence of DNA damage. (a–g) Synchronized TIG3(et) cells in G0 by serum starvation during 5 days with medium containing 0.5% FBS, then released in 10% FBS medium and treated with curcumin or infected with shp300-1 (right panel). Vehicle (0) or empty vector (−) as control. 1 μM aphidicolin-treated cells (aph) for 24 h were used as positive control. (a) Immunofluorescence of γH2AX and Hoechst staining to detect DNA. (b) Quantification of DNA breaks by comet assay. Mean value of tail moments from three independent experiments. Boxes correspond to 25–75 percentile, whiskers to 5–95 percentile and the line near the middle of the box marks the median (50th percentile). Statistical analysis was performed using the unpairedttest (***P<0.0001; NS, not significant). Immunoblot analysis with (c) whole cell extract with β-actin as loading control and (d) chromatin extract with H3 as loading control. (e) Cells were released in 10% FBS medium in presence or absence of curcumin and in presence or absence of 1 mM caffeine (Caff.). Cells were collected 72 h after release and analysed by FACS. Shown are the results of two independent experiments performed in duplicate. Error bars show the range. (f, g) Cells were released in 10% FBS medium in presence of curcumin or vehicle for 24 h and then co-treated with 1 μM of aphidicolin (aph) or vehicle as a control for 24 h. Immunofluorescence (f) and immunoblot (g) analysis performed after 24 h of co-treatment. (a,f) Scale bars are equal to 5 μm. As shown in Figure 4c , we observed a decrease of Cdc25B expression in curcumin-treated and p300kd cells. This result is consistent with the absence of DNA damage and DDR activation in curcumin-treated and p300kd cells. Furthermore, this could explain the G2/M phase cell cycle arrest. Finally, we showed that p300 HAT inhibition does not prevent DNA damage, when the DNA damaging agent aphidicolin is added, as observed by the presence of γH2AX foci in aphidicolin curcumin-treated cells ( Fig. 4f–g ). Our results show that SAHF formation during the S phase, triggered by the inhibition of p300 HAT activity, does not induce DNA damage and DDR activation, which is in agreement with the conserved distribution of the various replication patterns and the absence of variation of the median inter-origin distances, previously observed by molecular DNA combing ( Figure 3d,e ; Supplementary Fig. S5 ). Together, these results indicate that p300 HAT inhibition triggers a reset and an extended period for the timing of replication origin cluster activation for S-phase completion. Furthermore, this senescence, which is associated to a chromatin-dependent replication stress, does not generate DNA damage or stress-induced activation of dormant origins, as revealed by the absence of phosphorylation of CHK1 and CHK2. Figure 4: Inhibition of p300 HAT induces senescence in absence of DNA damage. ( a–g ) Synchronized TIG3(et) cells in G0 by serum starvation during 5 days with medium containing 0.5% FBS, then released in 10% FBS medium and treated with curcumin or infected with shp300-1 (right panel). Vehicle (0) or empty vector (−) as control. 1 μM aphidicolin-treated cells (aph) for 24 h were used as positive control. ( a ) Immunofluorescence of γH2AX and Hoechst staining to detect DNA. ( b ) Quantification of DNA breaks by comet assay. Mean value of tail moments from three independent experiments. Boxes correspond to 25–75 percentile, whiskers to 5–95 percentile and the line near the middle of the box marks the median (50th percentile). Statistical analysis was performed using the unpaired t test (*** P <0.0001; NS, not significant). Immunoblot analysis with ( c ) whole cell extract with β-actin as loading control and ( d ) chromatin extract with H3 as loading control. ( e ) Cells were released in 10% FBS medium in presence or absence of curcumin and in presence or absence of 1 mM caffeine (Caff.). Cells were collected 72 h after release and analysed by FACS. Shown are the results of two independent experiments performed in duplicate. Error bars show the range. ( f, g ) Cells were released in 10% FBS medium in presence of curcumin or vehicle for 24 h and then co-treated with 1 μM of aphidicolin (aph) or vehicle as a control for 24 h. Immunofluorescence ( f ) and immunoblot ( g ) analysis performed after 24 h of co-treatment. ( a,f ) Scale bars are equal to 5 μm. Full size image Senescence induction is independent of p53/p21 CIP1 /p16 INK4A Senescence growth arrest usually depends on the activation of the CDK inhibitors (p21 CIP1 and p16 INK4A ), components of the tumour-suppressor pathways governed by the p53 and retinoblastoma (pRB) proteins, respectively, and is generally associated with a G1 senescence cell cycle arrest [2] . However, the inhibition of p300 HAT activity led to G2/M senescence arrest within one cell cycle, which requires SAHF formation and S-phase progression, suggesting that increased expression of both proteins p21 CIP1 and p16 INK4A might not be directly involved in this senescence induction. To investigate whether this senescence growth arrest might be independent of the activation of p53/p21 CIP1 and p16 INK4A pathways, we treated TIG3(et) cells with stable knockdown of p16 INK4A , p21 CIP1 , p53 or in combination with curcumin. After 8 days of curcumin treatment, we observed, as previously shown, an induction of p21 CIP1 and p16 INK4A expression in the parental cells, but only the induction of p21 CIP1 in p16kd cell lines and only the induction of p16 INK4A in p21 CIP1 kd and p53kd cell lines ( Fig. 5a ). 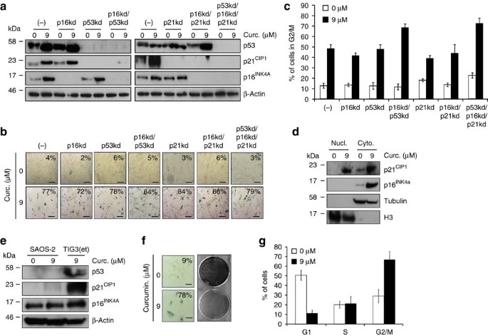Figure 5: Inhibition of p300 HAT activity induces a p53/p21CIP1/p16INK4A - independent induction of senescence. (a,b) TIG3(et) indicated knockdown cells and TIG3(et)/(–) for empty vector synchronized in G0 by serum starvation during 5 days with medium containing 0.5% FBS, then released in 10% FBS medium in presence of 9 μM of curcumin (Curc.) or vehicle (0) as control and analysed 8 days after release. (a) Immunoblot analysis with β-actin as loading control and (b) SA-β-gal activity. (c) Percentage of cells in G2/M phase analysed by FACS in TIG3(et) knockdown cell lines after 3 days of curcumin treatment. (d) Synchronized TIG3(et) cells in G0 by serum starvation during 5 days with medium containing 0.5% FBS, then released in 10% FBS medium in presence of 9 μM of curcumin (Curc.) or vehicle (0) as control and analysed 8 days after release. Nuclear (Nucl.) and cytoplasmic (Cyto.) fractions were analysed by western blot using H3 and tubulin as loading control for the nuclear and the cytoplasmic fractions, respectively. (e–g) Synchronized osteosarcoma SAOS-2 cell line in G0 by serum starvation during 5 days with medium containing 0.5% FBS, then released in 10% FBS medium in presence of 9 μM of curcumin or vehicle (0) as control. (e) Immunoblot analysis with β-actin as loading control and curcumin-treated TIG3(et) cells as immunoblot control, and (f) SA-β-gal activity (left panel) and coomassie staining (right panel) analysed 8 days after release. (g) Cell cycle distribution analysed by FACS after 3 days of curcumin treatment. (b,f) Percentage of SA-β-gal positive cells is indicated in insert. (c,g) Shown are the results of two independent experiments performed in duplicate. Error bars show the range. (b,f) Scale bars are equal to 40 μm. Strikingly, single or double knockdown of these genes did not prevent senescence induction by inhibition of p300 HAT activity, as observed by reduced proliferation, an increase in SA-β-Gal activity and SAHF formation ( Figure 5a,b ; Supplementary Fig. S6 ). Finally, TIG3(et) cells with simultaneously stable knockdown of p53, p16 INK4A and p21 CIP1 produced a similar result. Furthermore, we still observed a G2/M cell cycle arrest in these different TIG3(et) knocked-down cell lines ( Fig. 5c ), indicating that this specific cell cycle arrest is not triggered by upregulation of these CDK inhibitors. Because the accumulation of p21 CIP1 and p16 INK4A in curcumin-treated cells does not seem to be required for SAHF formation and senescence arrest, we hypothesized that these proteins might be inactivated or mislocalized in cells where p300 activity is inhibited. We performed nuclear and cytoplasmic cell fractionations and showed that p21 CIP1 and p16 INK4A accumulate primarily in the cytoplasm of curcumin-treated cells ( Fig. 5d ), suggesting that the induction of these proteins does not regulate the cell cycle but might have other functions [24] , [25] . Although we cannot exclude that the induction of p21 CIP1 and p16 INK4A might participate in an extra step for stabilizing the cell cycle arrest later in the senescence process, we can conclude that senescence induction by inhibition of p300 HAT activity is independent of the p53/p21 CIP1 and p16 INK4A pathways. To further demonstrate the efficiency of this senescence-inducing mechanism, we used the osteosarcoma SAOS-2 cancer cell line, that is p53- and pRB-deficient [26] . We were also able to induce premature senescence and specific G2/M cell cycle arrest in SAOS-2 curcumin-treated cell line in the absence of p53 and pRB pathway activation ( Fig. 5e–g ). Altogether, these results show that inhibition of p300 HAT is able to induce a p53/p21 CIP1 - and p16 INK4A -independent senescence-like growth arrest in normal and cancer cell lines. Figure 5: Inhibition of p300 HAT activity induces a p53/p21CIP1/p16INK4A - independent induction of senescence. ( a,b ) TIG3(et) indicated knockdown cells and TIG3(et)/(–) for empty vector synchronized in G0 by serum starvation during 5 days with medium containing 0.5% FBS, then released in 10% FBS medium in presence of 9 μM of curcumin (Curc.) or vehicle (0) as control and analysed 8 days after release. ( a ) Immunoblot analysis with β-actin as loading control and ( b ) SA-β-gal activity. ( c ) Percentage of cells in G2/M phase analysed by FACS in TIG3(et) knockdown cell lines after 3 days of curcumin treatment. ( d ) Synchronized TIG3(et) cells in G0 by serum starvation during 5 days with medium containing 0.5% FBS, then released in 10% FBS medium in presence of 9 μM of curcumin (Curc.) or vehicle (0) as control and analysed 8 days after release. Nuclear (Nucl.) and cytoplasmic (Cyto.) fractions were analysed by western blot using H3 and tubulin as loading control for the nuclear and the cytoplasmic fractions, respectively. ( e–g ) Synchronized osteosarcoma SAOS-2 cell line in G0 by serum starvation during 5 days with medium containing 0.5% FBS, then released in 10% FBS medium in presence of 9 μM of curcumin or vehicle (0) as control. ( e ) Immunoblot analysis with β-actin as loading control and curcumin-treated TIG3(et) cells as immunoblot control, and ( f ) SA-β-gal activity (left panel) and coomassie staining (right panel) analysed 8 days after release. ( g ) Cell cycle distribution analysed by FACS after 3 days of curcumin treatment. ( b,f ) Percentage of SA-β-gal positive cells is indicated in insert. ( c,g ) Shown are the results of two independent experiments performed in duplicate. Error bars show the range. ( b,f ) Scale bars are equal to 40 μm. Full size image p300 HAT was originally identified as a binding partner of the adenovirus early region 1A (E1A) [27] . p300 catalyzes the acetylation of all four core histones, and has been reported to acetylate several other proteins and itself [9] . p300 has been implicated in many different cellular functions, and gene mutations have been detected in human tumours, with loss-of-function point mutations found in colorectal, breast, ovarian, lung, gastric and pancreatic carcinomas, leading to the hypothesis that p300 might be a tumour suppressor gene [28] , [29] , [30] . Senescence can be triggered through either the activation of oncogenes or the loss of tumour suppressor gene, such as PTEN , RB1 or NF1 (refs 31 , 32 , 33 ). Our results revealed that loss of p300 HAT activity or p300 expression had the same effect on cellular senescence induction. The hypoacetylation of the histone H3/H4 and the increase of nucleosome density due to the histone chaperone complex HIRA/ASF1a-mediated nucleosome deposition are among the earliest step of SAHF formation [7] . Interestingly, the inhibition of p300 HAT activity by specific inhibitors or shRNA induces the immediate and global hypoacetylation of histones H3 and H4, followed by a subsequent S-Phase-initiated SAHF formation ( Figs 1 and 3 ), suggesting that p300 HAT inactivation could be implicated in the first step of SAHF formation. This hypothesis is consistent with the decrease in SAHF, observed when HMGA1 (one of the first proteins involved in SAHF formation), was dowregulated in addition to p300 inhibition ( Fig. 2f,g ). This is further corroborated by the strong decrease in p300 expression in oncogene-induced and replicative senescence ( Supplementary Fig. S1 ), suggesting that it might constitute a common event in different types of senescence in primary fibroblasts. DNA replication is a tightly regulated process that was previously described to be altered in senescence. In particular, expressing an activated oncogene in normal human cells leads to a first hyper-proliferation phase. However, our results showed that p300 HAT inhibition-induced senescence is associated rather with a decrease in cell cycle progression. Moreover OIS is related to an over-replicative phase with an increased number of stress-induced active replicons leading to alterations in DNA replication fork progression and a subsequent robust DDR [3] , [4] . Strikingly, although we showed that p300 HAT inhibition-induced senescence leads to a marked slowdown of the global replication fork velocity, we did not detect any significant changes in the mean number of active replicons related to replication stress ( Fig. 3d,e ; Suppementary Fig. S5 ). Furthermore, we did not observe any activation of DDR or induction of DNA damage ( Fig. 4 ). The absence of DDR was also described in another type of senescence induction, Pten-loss-induced cellular senescence, but in this case, cellular senescence occurred in the absence of DNA replication [34] , which is in contrast to the senescence induction by p300 HAT inactivation, in which DNA replication is required for SAHF formation and cell cycle arrest ( Fig. 2e ). These results highlight the difference between previously described mechanisms for senescence induction and this new type of senescence regarding the presence of DNA damage and activation of supplementary replicons. In this report, we described, for the first time, the link between senescence induction and the alteration of replication timing ( Fig. 3g ). A correlation between replication time, chromatin structure and transcriptional activity has long been observed, but recent genome-wide studies revealed that a large fraction of the genome is subjected to dynamic changes during development, allowing the establishment of cell-type specific replication timing profiles [35] , [36] , [37] . Replication timing is therefore thought to represent a mitotically stable cell-type specific feature of chromosomes. Many studies suggest that replication timing can affect chromosome condensation, sister chromatid cohesion, and genome stability [38] , promoting abnormal replication timing control as clinical marker in cancers. The level of histone acetylation is a mark that distinguishes early- and late-replicating regions. For instance, in early S phase, histones H3 and H4 embedded in chromatin are generally hyperacetylated, whereas in late S phase they are hypoacetylated, regulating the time of replication origin firing [14] , [15] . Because the replication time is coordinately regulated at the level of large megabase-sized domains, a change in replication timing would rapidly transmit a change in chromatin state to entire chromosomal domains, that could be responsible for the formation of SAHF and then to the senescence-induced growth arrest. The immediate and global histone hypo-acetylation triggered by p300 HAT inactivation, promoting the formation of heterochomatin alters the replication timing marks, leading to a doubling of S-phase length. Although not related to DDR activation, these alterations challenging chromosome condensation are likely to be sensed as a sudden onset of stress, such as is observed in osmotic shock or hypothermia [39] . A rapid response system, that does not require transcription or translation could then quickly trigger a block of the cell cycle in G2/M, involving Cdc25B [40] . Indeed, G1 cell cycle arrest is a common feature of cellular senescence and occurs progressively over multiple cell cycles [2] , related to accumulation of genomic alterations that threaten genome stability. Interestingly, the inhibition of p300 HAT activity leads to an atypical G2/M cell cycle arrest that occurs within a single cell cycle and requires SAHF formation during the preceding S-phase ( Fig. 2 ). Furthermore, we observed a decrease in Cdc25B, a dual specificity phosphatase, ( Fig. 4c ) that controls the G2/M phase checkpoint by activating CDK1-Cyclin B activity and was shown to be a specific target of a nongenotoxic stress checkpoint [23] . Interestingly, Cdc25B is degraded by the ubiquitin-proteasome pathway and depends on the F-box protein β-TrCp. Thomas and colleagues established a stabilized mutant of Cdc25B, which can not interact with βTrCP, increasing the half-life of the protein [41] . It might be interesting to overexpress this stabilized mutant to see whether it could impair the G2/M cell cycle arrest induced by p300 inhibition. But, assuming that different types of chromatin, assembled at the replication fork at different times during S-phase, can also influence gene expression [14] , [42] , we cannot exclude that SAHF formation due to changes in chromatin status might also change gene expression, which may also participate to the establishment of the senescent phenotype. Senescence growth arrest usually relies on the activation of the CDK inhibitors (p21 CIP1 and p16 INK4A ), components of the tumour-suppressor pathways governed by the pRB proteins, respectively. Interestingly, although we observed increased expression of these proteins, we demonstrated that p300 HAT inhibition-induced senescence is independent of p53, p21 CIP1 and p16 INK4A ( Fig. 5 ). Moreover, we showed that p21 CIP1 and p16 INK4A accumulate primarily in the cytoplasm of p300 inhibited cells, suggesting that the induction of these proteins does not regulate the cell cycle but might have other cellular functions such as previously identified in apoptosis resistance or metastatic inhibition [24] , [25] . Furthermore, the lack of a requirement of p53, which is usually linked with DDR activation, reinforces our observation that p300 HAT inhibition-induced senescence occurs in the absence of DNA damage. Senescence has been shown to inhibit tumour progression in vivo [1] , thus the induction of senescence may represent a new alternative strategy to eradicate cancer [43] . Unfortunately, senescence usually relies on the activation of p53 and pRB tumour suppressor pathways that are often mutated or lost in tumours [44] , reducing the number of cancer types treatable by senescence induction. Furthermore, senescence induction by drugs or oncogenes often triggers a DDR that might challenge the genome integrity of cells. Interestingly, we were able to induce senescence in the osteosarcoma SAOS-2 cancer cell line, that is p53- and pRB-deficient, by treating them with a low dose of curcumin that inhibits p300, and does not trigger the DDR, potentially opening a new window for the treatment of tumours that are resistant to classical chemotherapy and that carry mutations in the p53 and/or pRB pathways ( Fig. 5e–g ; Supplementary Fig. S6 ). Curcumin, that is found in the diet, has already proven to be useful in chemoprevention for colorectal [45] and pancreatic cancer [46] . Overall, our results reveal a new and unexpected mechanism for senescence induction, by a chromatin-dependent alteration of S-phase progression, unrelated to genomic alterations. It may occur within only one cell cycle, independently of the activation of p53/p21 CIP1 and p16 INK4A /pRB pathways, but depends on SAHF formation and progression through S phase, providing new insights into the control of S-phase progression by p300. Interestingly, this new senescence-induced state, initiated by chromatin deacetylation, is also recapitulated by curcumin, a drug commonly found in the diet. These results illustrate a possible epigenetic control of senescence in aging, and also reveal unanticipated targets and mechanisms controlling the chromatin state that might be specifically triggered as an alternative strategy to treat proliferation disorders without generating further DNA damage. Reagents pBABE-puro-RAS V12 and pRetroSuper-p21 CIP1 were a kind gift from Dr. D. Peeper (The Netherlands Cancer Institute, Amsterdam). pSin-puro-miR30-HMGA1 was a kind gift from Dr. M. Narita (Cancer Research UK, Cambridge). pLKO-p300 with the following shRNA sequences No. 1 CCTCACTTTATGGAAGAGTT sequences, No. 2 GCCTTCACAATTCCGAGACAT are from Openbiosystem. pMKO.1-puro-p53 (plasmid 10672) was purchased from Addgene. Anti-p21 (C-19), anti-p16 (C-20), anti p53 (DO1), anti-minichromosome maintenance protein 7 (H-300), anti-PCNA (FL-261), anti-Cdc25B (C-20) and anti-CHK1 (G-4) were purchased from Santa-Cruz; Anti- histone H3K9me3 (Ab8898), anti-H3K56ac (ab76307), anti-H4 (ab52178) and anti-H3 (Ab1791) from Abcam; anti- HP1γ (2-MOD-166-as) were purchased from Euromedex; and anti-β-actin (H9537) and anti-H4ac (06-866) from Millipore; anti-p300 (05-257) were purchased from Upstate. Anti-Ras (610002) was purchased from BD laboratories and anti-CHK2 (2662), Phospho-CHK2 (thr68) (2661), Phospho-p53 (ser15) (9287) and Phospho-CHK1 (ser345) (2341) were purchased from Cell Signaling. Finally, anti-γH2AX (07-219) and anti-tubulin (T6199) were purchased from Sigma. HMGA1 antibody was kindly provided by Dr. M. Narita (Cancer Research UK, Cambridge). All the antibodies were used at 1/1,000 dilution except anti-H3 and anti-β-actin that were used at 1/10,000 dilution, Curcumin (81025.1) was purchased from Cayman Chemical; aphidicolin (A0781), mimosine (M0253) and caffeine (C0750) from Sigma; CTPB (ALX-420-033-M005) from Coger. C646 and C37 were a kind gift from Dr. P Cole (Johns Hopkins University School of Medicine, Baltimore). Cell culture TIG3 and BJ human diploid fibroblasts expressing the ecotropic receptor and hTERT TIG3(et), BJ(et), TIG3(et)/p16kd, TIG3(et)/p53kd and Phoenix cells were a kind gift from Dr. D. Peeper (The Netherlands Cancer Institute, Amsterdam). The osteosarcoma SAOS-2 cell line was a kind gift from Dr. O. Delattre (Institut Curie, Paris). HDF1 human diploid fibroblasts were a kind gift from Dr. J. Piette (IGMM, Montpellier, France). Cells were cultured in DMEM (Life technologies) supplemented with 10% FBS (Greiner bio-one), 2 mM l-glutamine, 100 units per ml penicillin and 0.1 mg ml −1 streptomycin (all Gibco). In some experiments, TIG3(et) cells were synchronized in G0 phase by serum starvation for 5 days with medium containing 0.5% FBS, then cells were re-seeded at a density 10 6 cells per 10 cm dish. The following day, cells were released from cycle arrest in 10% FBS medium in the absence or presence of specific drugs. For cell cycle profile studies, cells were labelled with 10 μM BrdU for 3 h then fixed in 70% Et-OH for at least 4 h at 4°C. Cell pellets were washed with PBS then treated with RNAse A (0.5 mg ml −1 ) for 30 min at 37 °C, then washed again with PBS. Pellets were treated with 5 M HCl/H 2 O/0.5% triton for 20 min at room temperature, then washed with Tris 1 M pH 7.5. Pellets were resuspended with primary and secondary antibodies in PBS/0,2% tween-20/1% BSA for 45 min and washed with PBS/0.2% tween-20. Finally, pellets were resuspended with Propidium Iodide (20 μg ml −1 ) in PBS and analysed by FACS (Facscalibur II). For the production of lentiviruses, 293 T cells were transfected by the calcium-phosphate method using 20 μg of transfer vector pLKO-p300, 15 μg of packaging vector psPAX2 (addgene) and 6 μg of envelope vector pMD2.G (addgene). Lentiviruses were collected 24 and 48 h after transfection and filtered through a 0.45-μM filter. For the production of retroviruses, Phoenix cells were transfected by the calcium-phosphate method using 25 μg of transfer vector pMKO.1-puro-p53 or pBABE-puro-RAS V12 or pRetroSuper-p21 CIP1 . Retroviruses were collected 24 and 48 h after transfection and filtered through a 0.45 μM filter. For SA-β-gal activity, cells were washed in PBS, fixed for 5 min in 2% formaldehyde/0.2% glutaraldehyde, washed and incubated at 37 °C with fresh SA-β-gal stain solution: 1 mg ml −1 of X-gal/40 mM citric acid/sodium phosphate, pH 6.0/5 mM potassium ferrocyanide/5 mM potassium ferricyanide/150 mM NaCl 2 /2 mM MgCl 2 (ref. 47 ) and monitored as the per cent of cells with SA-β-gal staining divided by the total number of cells in 10 independent fields. For coomassie staining, 2×10 5 cells were seeded into 6-well plates, and fixed and stained 8–12 days after the beginning of the treatment [48] . Immunofluorescence 2×10 4 cells were plated on LabTek slides (Nalge Nunc International) and left in complete medium for the indicated time, washed in PBS, fixed in 4% PBS-buffered formaldehyde for 15 min, permeabilized in 0.2% tritonX100-PBS, blocked in PBS–BSA 2% for 1 h, incubated with indicated primary antibodies for 45 min, and with fluorescent secondary antibody for 30 min and counterstained with Hoechst 33342 (Invitrogen). EdU staining was performed according to the manufacturer's instructions (Invitrogen). SAHF detection was generally examined by Pan-DNA staining dye Hoeschst (1 mg·ml −1 ), and extra markers such as H3K9Me3 and HMGA1 were also detected in some experiments [5] , [6] , [7] . The percentage of γ-H2AX positive cells was calculated from cells containing at least 5 foci in their nucleus divided by the total number of cells in 10 independent fields. The fluorescent Comet assay (Trevigen) was performed in accordance with the manufacturer's instructions. Protein extracts For the whole cell extract, cells were lysed in RIPA buffer (1% NP40, 1% SDS, 0.5 DOC, 50 mM Tris–HCl pH 8, 2 mM EDTA). For the chromatin fraction extract, cells were washed with PBS, resuspended in Chelsky buffer (10 mM Tris–HCl pH 7.5, 10 mM NaCl, 3 mM MgCl 2 , 30 mM sucrose) and centrifuged for 15 min at 1,500 g . The pellet was lysed with Chelsky buffer containing 0.5% NP-40 and centrifuged for 15 min at 1,500 g . The pellet was then resuspended in Chelsky buffer, centrifuged for 15 min at 3,000 g through a 0.7 M sucrose cushion and then resuspended in 1× sample buffer. For nuclear/cytoplasmic protein extraction, cells were washed and scrapped in ice-cold PBS. The pellet was washed in wash buffer (10 mM HEPES pH 7.9, 20 mM KCl, 2 mM MgCl 2 , 0.1 mM EDTA pH 7), centrifuged for 1 min, lysed in cytoplasmic extraction buffer (10 mM HEPES pH 7.9, 10 mM KCl, 2 mM MgCl 2 , 0.1 mM EDTA pH 7, 0.2% NP40) supplemented with protease inhibitor cocktail and centrifuged to removed cellular debris. Pelleted nuclei were resuspended in nuclear extract buffer (20 mM HEPES pH 7.9, 0.63 M NaCl, 1.5 mM MgCl 2 , 0.2 mM EDTA pH 7, 25% glycerol) supplemented with protease inhibitor cocktail, incubated for 30 min at 4 °C, centrifuged for 30 min at 14,000 and the protein amounts were quantified using Bradford method. DNA combing For replication timing studies, TIG3(et) cells were synchronized in G0 phase by serum starvation during 5 days with medium containing 0.5% FBS, then re-set up at 10 6 cells per 10-cm dish. The day after, cells were released in 10% FBS medium and pulse labelled for 3 h with 25 μM IdU followed by a 3-h chase with thymidine to label DNA at the early S phase. Cells were resynchronized by serum starvation for 5 days and re-set up on glass slides. Then, arrested cells were released in 10% FBS in presence of 9 μM curcumin and pulse labelled for 3 h with CldU in early, middle or late S phase, according to the results of S-phase length obtained in Supplementary Figure S4 . Cells were collected and treated for DNA combing. For specific measurement of replication fork velocity and inter-origin distances, cells were successively labelled for 15 min with 20 μM IdU and for 30 min with 100 μM CldU and collected for DNA combing. DNA combing was performed as followed. Briefly, cells were collected after the CldU labelling and embedded in agarose plugs (about 1.5×10 5 cells/plugs). DNA was stained with YOYO-1 (Invitrogen), and resuspended in 50 mM MES (pH 5.7) after digestion of the plugs with agarase (Biolabs). DNA fibres were stretched on silanized coverslips. Combed DNA fibres were denatured for 30 min with 0.5N NaOH. IdU was detected with a mouse monoclonal antibody (BD44 Becton Dickinson; 1:20 dilution) and a secondary antibody coupled to Alexa 546 (A21123, Invitrogen, 1:50 dilution). CldU was detected with a rat monoclonal antibody (BU1/75, AbCys; 1:20 dilution) and a secondary antibody coupled to Alexa 488 (A11006, Invitrogen; 1:50 dilution). DNA was detected with an anti-ssDNA antibody (MAB3034, Euromedex; 1:100 dilution) and an anti-mouse IgG2a coupled to Alexa 647 (A21241, Invitrogen, 1:50 dilution). Then immunodetection of DNA fibres were analysed on a Leica DM6000B microscope equipped with a CoolSNAP HQ CCD camera (Roper Scientifics). Data acquisition was performed with MetaMorph (Universal Imaging). Box-and-whiskers graphs were plotted with Prism v5.0 (GraphPad Software). For all graphs, whiskers correspond to 5–95 percentile and the line near the middle of the box marks the median (50th percentile). Data not included between the whiskers are plotted as outliers (dots). Statistical analysis was performed in Prism v5.0 (GraphPad) using the unpaired t test. How to cite this article: Prieur, A. et al . p53 and p16 INK4A independent induction of senescence by chromatin-dependent alteration of S-phase progression. Nat. Commun. 2:473 doi: 10.1038/ncomms1473 (2011).